Non-canonical activation of OmpR drives acid and osmotic stress responses in single bacterial cells Unlike eukaryotes, bacteria undergo large changes in osmolality and cytoplasmic pH. It has been described that during acid stress, bacteria internal pH promptly acidifies, followed by recovery. Here, using pH imaging in single living cells, we show that following acid stress, bacteria maintain an acidic cytoplasm and the osmotic stress transcription factor OmpR is required for acidification. The activation of this response is non-canonical, involving a regulatory mechanism requiring the OmpR cognate kinase EnvZ, but not OmpR phosphorylation. Single cell analysis further identifies an intracellular pH threshold ~6.5. Acid stress reduces the internal pH below this threshold, increasing OmpR dimerization and DNA binding. During osmotic stress, the internal pH is above the threshold, triggering distinct OmpR-related pathways. Preventing intracellular acidification of Salmonella renders it avirulent, suggesting that acid stress pathways represent a potential therapeutic target. These results further emphasize the advantages of single cell analysis over studies of population averages. Eukaryotes tightly regulate cytoplasmic pH and osmolality to be isosmotic and pH balanced with blood (290 mOsm Kg −1 , pH 7.35–7.45). In contrast, Gram-negative bacteria can undergo large changes in osmolality (up to 1800 mOsm Kg −1 ) [1] and endure a substantial reduction in cytoplasmic pH (to 5.5 or lower) [2] . E. coli is known to be capable of colonizing the gastrointestinal tract by its ability to grow over a wide pH range (4.5–9.0) [3] , [4] , [5] , yet E. coli and S. Typhimurium are considered to be neutralophiles, i.e., they maintain their intracellular pH (pH i ) between 7.5 and 7.7 [6] . Previous studies report that in response to acid stress, E. coli rapidly acidifies and then recovers [7] , but the essential components of this recovery process remain poorly understood. Furthermore, many intracellular pathogens survive within a membrane-bound acidic compartment inside macrophages. We recently placed a novel FRET DNA biosensor (the “I-switch”) inside S. Typhimurium and measured its intracellular pH in the macrophage vacuole [2] . Surprisingly, the S. Typhimurium cytoplasm acidified in a process that was dependent on the EnvZ-OmpR signal transduction system and acidification was essential for S. Typhimurium virulence. Because our observation of prolonged acidification of S. Typhimurium [2] was in conflict with previous studies in E. coli [7] , we set out to re-examine pH regulation in E. coli and S . Typhimurium. We labeled S. Typhimurium in culture with either the I-switch, or with the fluorescent pH indicator BCECF-AM. Single cell analysis using either probe indicated that bacteria fail to recover from acid shock, but maintain their cytoplasmic pH to be slightly less acidic (~0.3–0.6 pH units) than the extracellular pH (pH e ). Acidification is dependent on the response regulator OmpR, known to be involved in the acid tolerance response in S. Typhimurium [2] and in osmoregulation of outer membrane proteins OmpF and OmpC (see ref. [8] for a review). In response to both acid and osmotic stress, the cytoplasm acidifies in an OmpR-dependent manner, although the pathways are distinct. The pathways are distinct because the intracellular pH is more acidic in response to acid stress compared to osmotic stress. Under acidic conditions, the sensor kinase EnvZ is activated by increased helicity of a disordered region that surrounds the phosphorylated histidine [9] . This activation step promotes interaction with OmpR [10] , driving an active OmpR conformation. This is evident by an EnvZ-dependent, phosphorylation-independent increase in OmpR dimer formation, which facilitates high-affinity DNA binding and alteration of gene expression (usually repression). An EnvZ mutant that is unable to interact with OmpR [10] fails to acidify in response to both acid and osmotic stress. OmpR-driven repression is independent of OmpR phosphorylation and thus, is non-canonical [11] . An acid-dependent increase in the affinity of OmpR binding to DNA at the ompC and cadB/A promoters was identified by atomic force microscopy (AFM). In contrast, genes that are activated by OmpR (e.g., ompF and ompC ), require OmpR phosphorylation to create a productive interaction with RpoA, the alpha subunit of RNA polymerase [12] . Herein, we establish that pHluorin, when expressed as an arabinose-inducible, plasmid-encoded, pH-sensitive GFP, is heterogeneous with respect to its expression in single cells and thus, it is not a good indicator for pH measurements in bacteria. Many previous studies also used sodium benzoate as a clamping agent that was reported to equilibrate the internal pH i with the external pH e . Comparison of the standard curve of cells clamped using the ionophore nigericin and generated from the I-switch or BCECF, with cells clamped using the weak acid sodium benzoate dramatically illustrates that sodium benzoate is a poor choice as a clamping agent. Lastly, we provide evidence that the E. coli strain MC4100 responds differently to extracellular acid or osmotic stress compared to the probiotic Nissle strain [13] , [14] and to MG1655, a sequenced strain [15] . It appears that the large deletions that occurred during the construction of MC4100 for making lacZ transcriptional fusions made it a poor strain for studying E. coli physiology [16] . Thus, we now have a radically different view of pH regulation in Gram-negative bacteria that centers on an acid-sensitive conformational switch in OmpR that facilitates repression of acid response genes to maintain an acidic cytoplasm. Our results also implicate acidification as essential for virulence and we can now identify potential targets for therapeutic intervention. Lastly, this study identifies a pH threshold in bacteria, below which OmpR phosphorylation is low, but dimerization is high and DNA binding is driven by an acid-dependent conformational change in OmpR. Unique genes are expressed above and below this threshold, allowing integration of osmotic and acid stress signals. In this study, we establish OmpR as a global regulator of acid and osmotic stress in S. Typhimurium and E. coli . OmpR represses distinct sets of genes based on the intracellular pH threshold (~6.5) that neutralize the bacterial cytoplasm, thus enabling acidification. The response to acid stress involves repression of lysine decarboxylation, whereas the osmotic stress response in Salmonella works through repression of rpoS , activating an oxidoreductase that produces protons. In E. coli , repression of ornithine decarboxylation acidifies the cytoplasm during osmotic stress. OmpR acts non-canonically, in that it depends on its kinase EnvZ, but phosphorylation is not required. Lastly, we highlight the importance of single cell imaging over population averages and explain why our results differ from previous studies. The EnvZ-OmpR acid stress response acidifies the cytoplasm We previously determined that S . Typhimurium reduced its intracellular pH in response to external acid stress in an OmpR-dependent manner [2] , in contrast to previous studies in E. coli that reported a rapid recovery within minutes [17] , [18] . We set out to reconcile these differences by measuring the cytoplasmic pH and recovery of S. Typhimurium and E. coli immediately following an external acid shift. In S . Typhimurium, the cytoplasmic pH decreased from 6.80 to 6.35 within 5 min at pH e 5.6 and reached a plateau value of 6.15 after 90 min (Fig. 1a , b). In contrast, the cytoplasm remained unchanged (pH 6.80) when incubated at pH e 7.2. No decrease in cytoplasmic pH was observed in an ompR null strain of S . Typhimurium (pH 6.75), confirming the existence of an OmpR-dependent acidification process [2] . In E. coli , the initial pH of the cytoplasm was slightly higher (pH 7.13) compared to S . Typhimurium (pH 6.80), but a comparable decrease in pH i from 7.13 to 6.55 occurred during 90 min exposure to acid stress (Fig. 1c, d ). In an ompR null strain of E. coli , intracellular pH did not decrease in response to extracellular acid stress, establishing OmpR as a regulator of acid stress in both S . Typhimurium and E. coli (Fig. 1 and refs. [2] , [19] ). Fig. 1 OmpR drives intracellular acidification in response to acid stress. a – d S . Typhimurium and E. coli cultures were incubated with 20 µM BCECF for 60 min before imaging. Representative epifluorescence ratio images (R 488/440 ) of emission channel 525 nm upon 488 nm excitation and 440 nm excitation were obtained for wild type, an ompR null mutant, an ompR /cad BA null strain, a cadBA null strain, and a cadBA over-expressed strain of a S . Typhimurium and c E. coli incubated at either acidic pH e (5.6) or neutral pH e (7.2) or at pH e (7.2) plus 15% (w/v) sucrose. Using ImageJ software, ratio images were color coded with blue (ratio = 0.1) to white (ratio = 1). Scale bar, 3 µm. A plot of the intracellular pH of 50 cells of wild type and mutants of b S . Typhimurium and d E. coli at each indicated time point. Error bars represent the mean ± s.e.m. ( n = 3). The complete graphs including all strains in b , c are in Supplementary Fig. 2 . Repression of the cad operon was not responsible for intracellular acidification during osmotic stress in S . Typhimurium and E. coli Full size image Acidification via OmpR repression of lysine decarboxylation In S . Typhimurium, OmpR prevents recovery from acidification by repressing cadC/BA . CadA encodes a lysine decarboxylase, CadB encodes a lysine/cadaverine antiporter, and CadC encodes a transcriptional regulator. We performed quantitative real-time PCR (qRT-PCR) with E. coli and observed an increase in transcript levels of cadB (4.5-fold) and cadA (3-fold) in the ompR null mutant, suggesting that E. coli OmpR also functions as a repressor at this locus (Supplementary Fig. 1a ). OmpR repression resulted from direct interaction at the cadC/BA locus, based on electrophoretic mobility shift assays (EMSAs) (Supplementary Fig. 1b ). OmpR did not bind at cadA (Supplementary Fig. 1b ), suggesting that cadB and cadA are co-transcribed, as we also observed in S . Typhimurium [2] . To determine whether cadC/BA repression was sufficient to prevent recovery from acid stress, we measured the response of an ompR / cadBA null strain, a cadBA null strain, and a cadBA over-expressed strain of E. coli exposed to similar acid stress. As with S . Typhimurium (Fig. 1a , b and ref. [2] ), OmpR was no longer required for cytoplasmic acidification when cadBA was eliminated, indicating that the CAD system was the main pathway for recovery from acidification between pH 6.1 and 6.5 (Fig. 1c, d ). Furthermore, when cadBA was over-expressed in E. coli , OmpR was unable to repress cadC/BA , and the cytoplasm was neutralized. Overexpression of additional decarboxylases, such as glutamate ( gadBA ), arginine ( speA ), and S-adenosylmethionine decarboxylase ( speD ), during acid stress did not neutralize the pH i (Supplementary Fig. 1c, d ), suggesting that cadBA was the major system that eliminated protons upon acid stress in E. coli over the approximate pH i range of 6.1–6.5. This was not surprising, since the glutamate and arginine decarboxylation systems exhibit much lower pH optima (pH 4 and 5, respectively) [20] , compared to lysine (pH 6.1–6.5) [21] , S-adenosylmethionine decarboxylase (pH 7.4) [22] and ornithine decarboxylase systems (pH 7.0) [23] . Furthermore, the pH i response of the cadBA null strain was similar to the wild type (Fig. 1 ). Thus, in both S. Typhimurium and E. coli , OmpR directly repressed cadC/BA to enable cytoplasmic acidification under acid stress. Osmotic stress acidifies S. Typhimurium and E. coli EnvZ has been described as an osmosensor, as high osmolality activates OmpR to differentially upregulate ompC and repress ompF (reviewed in ref. [8] ). Since EnvZ senses and responds to a concentrated cytoplasm [2] , [9] , we hypothesized that the cytoplasm might acidify during osmotic stress, indicating that EnvZ is actually functioning as a pH sensor. Using sucrose as the osmolyte, addition of 15% sucrose (w/v; 787 mOsm Kg −1 ) to the medium at pH e 7.2 led to a decrease in the pH i of S . Typhimurium from 6.80 to 6.45 (Fig. 1a, b ). In contrast, the ompR null strain remained near-neutral pH i , decreasing by <0.1 pH unit to 6.75 (Fig. 1a, b ). A similar decrease was evident in E. coli , where osmotic stress reduced the pH i from 7.13 to 6.75. The pH i of the ompR null E. coli strain did not decrease in response to sucrose-induced osmotic stress and remained at pH i 7.1 (Fig. 1c, d ). Thus, in both S. Typhimurium and E. coli , increasing external osmolality stimulated a prolonged, OmpR-dependent intracellular acidification (Fig. 1 ). Osmolyte-induced acidification is distinct from acid stress Overexpression of CAD did not protect S . Typhimurium or E. coli from acidification by osmotic stress (Fig. 1 ). Furthermore, elimination of cadB/A in an ompR null strain did not restore intracellular acidification at high osmolality in both S. Typhimurium (Fig. 1a, b and Supplementary Fig. 2a ) and E. coli (Fig. 1c, d and Supplementary Fig. 2b ), suggesting osmotic stress and acid stress pathways were distinct. However, osmolyte-driven intracellular acidification was sufficient to trigger virulence gene expression of Salmonella pathogenicity island 2 (SPI-2), as evidenced by ssrB transcription and effector SseJ secretion (Supplementary Fig. 3a, b ). To identify OmpR targets in response to acid stress, we performed a microarray-based expression analysis and compared the transcriptome of ompR null strains with wild-type strains of S. Typhimurium and E. coli during acid or osmotic stress (see data availability for full results through the GEO). In our S . Typhimurium microarray, the alternate sigma factor rpoS was upregulated 4.4-fold in the absence of ompR . RpoS was implicated in the acid-inducible exponential-phase acid tolerance response (ATR) of S . Typhimurium [24] , [25] , [26] and was essential for survival under acid stress [27] , [28] . In agreement with the upregulation observed by microarray, the rpoS transcript was up 4.8-fold in the ompR mutant (Fig. 2a ), suggesting that OmpR functions as a repressor at rpoS . Furthermore, the rpoS over-expressed strain maintained near-neutral pH i (6.8) in response to osmolytes, but was fully capable of cytoplasmic acidification by acid stress (Fig. 2b, c and Supplementary Fig. 4 ). Thus, the responses to acid stress and osmotic stress were distinct. Similarly, in the absence of rpoS , OmpR was not required for intracellular acidification at high osmolality (Fig. 2b, c and Supplementary Fig. 4 ). In response to acid stress, OmpR repressed the cadC/BA operon to maintain an acidic cytoplasm, whereas at high osmolality, an rpoS -dependent pathway was involved in S . Typhimurium acidification (Figs. 1 and 2 ). OmpR acted directly at rpoS , as determined by EMSAs with purified OmpR protein (Fig. 2d ), i.e., OmpR directly repressed rpoS transcription at high osmolality. Fig. 2 Osmotic stress acidifies S. Typhimurium via OmpR repression of rpoS . a mRNA levels of rpos and ssrA (a positive control) genes were determined by qRT-PCR from wild-type and ompR null strains of S . Typhimurium grown at high osmolality. Fold expression changes in the ompR null strain was compared to the wild-type level and plotted. The error bars represent the mean ± s.d. ( n = 6). In the ompR null strain, rpoS transcription was increased, suggesting OmpR repression. b Representative images of R 488/440 are shown after 5 and 90 min incubation at pH e 7.2 or pH e 7.2 in the presence of 15% (w/v) sucrose (high osm) of wild type, an ompR / rpoS null strain, an rpoS null strain, and an rpoS over-expressed strain of S . Typhimurium. Scale bar, 3 μm. c A plot from 50 cells of the R 488/440 ratios of various mutants of S . Typhimurium at indicated times. Symbols represent the mean ± s.e.m. ( n = 3). d An EMSA examined the interaction between OmpR and rpoS . OmpR was incubated with 10 fmol of biotin end-labeled rpoS . Lane 1.7* contained 100-fold excess unlabeled DNA Full size image To identify rpoS targets involved in intracellular acidification, we examined the microarray results for candidate targets that were downregulated in the ompR null strain and were known to be rpoS -dependent. We identified yghA , encoding a putative oxidoreductase, which was down 39-fold in the ompR null strain at high osmolality compared to the wild-type S. Typhimurium. This was confirmed by qRT-PCR, which indicated comparable downregulation of a yghA transcript (32-fold) in the ompR null strain, as well as in the rpoS over-expressed strain (26-fold), implicating RpoS as a repressor of yghA (Fig. 3a ). In contrast, in E. coli , YghA was not involved in osmotic stress-driven acidification, as yghA levels of the wild type and an ompR null strain were comparable (Fig. 3b ). As an oxidoreductase, YghA is predicted to oxidize NADH to liberate H + , leading to cytoplasmic acidification. In the absence of YghA, the S. Typhimurium cytoplasm would fail to acidify, due to a reduction in acid production. The pH i of a yghA null strain was 6.8 (i.e., not acidified) and thus, OmpR was no longer required to repress rpoS (Fig. 3c, d ). This result suggests a mechanism whereby OmpR relieves rpoS- dependent repression of yghA (which would be activating), to produce and maintain an acidified cytoplasm in response to osmotic stress. Furthermore, when yghA was over-expressed, the pH of the cytoplasm decreased to 6.45. In contrast, the ompR/rpoS/yghA null strain maintained near-neutral pH i (Fig. 3c, d ). OmpR did not bind directly to the yghA promoter, as evident from the EMSA (Fig. 3e ). This result was further supported by AFM imaging, and the relative height distribution histogram (Fig. 3f ). Instead, OmpR directly repressed rpoS transcription (Fig. 2 ), which increased yghA transcription (Fig. 3a, c, d ). Fig. 3 OmpR relieves RpoS repression of yghA during osmotic stress. a mRNA levels of yghA at pH e 7.2 in the presence of 15% sucrose (w/v) were determined by qRT-PCR from wild type, an ompR null strain, an rpoS over-expressed strain, and an ompR/rpoS null strain of S . Typhimurium. Fold expression changes were compared to the wild-type level. Error bars represent the mean ± s.d. ( n = 6). b mRNA of yghA at pH e 7.2 in the presence of 15% sucrose (w/v) of an E. coli ompR null strain was compared to the wild-type level. c Representative images of R 488/440 are shown after 5 and 90 min incubation at pH e 5.6, or pH e 7.2 + 15% (w/v) sucrose of a yghA null strain, an ompR / rpoS null strain, an ompR/rpoS/yghA null strain, and an ompR null strain of S. Typhimurium with yghA over-expressed. Scale bar, 3 μm. d Plot of the R 488/440 ratios of various mutants of S. Typhimurium at each indicated time. Data set is represented as the mean ± s.e.m. ( n = 3). The complete graph, including all strains is in Supplementary Fig. 4 . e EMSAs were performed with biotin end-labeled yghA and OmpR. f AFM images of yghA 700 from S . Typhimurium with 30 nM OmpR at either acid pH (6.1) or neutral pH (6.8). g Relative height distribution histogram of the yghA promoter complexed with 30 nM OmpR at either acidic or neutral pH Full size image Measurements of NAD + /NADH were consistent with these results (Supplementary Fig. 5a, b ). In the wild-type strain, yghA transcription increased 32-fold compared to an ompR null strain. Intracellular levels of NAD + in the wild type (52.3 nM) or an ompR/rpoS (51.3 nM) null strain were higher than an ompR null strain (29.6 nM), a yghA null strain (37.3 nM) or an ompR / yghA / rpoS (35.6 nM) null strain grown at high osmolality (Supplementary Fig. 5a, b ). Overexpression of yghA in an ompR null background completely restored intracellular NAD + to wild-type levels (49.6 nM). Increased NAD + levels were only observed at high osmolality and not during acid stress, further emphasizing the distinct responses to acid and osmotic stress. OmpR-dependent acidification occurs at high osmolality Microarray analysis comparing the wild-type and ompR null E. coli strains indicated that decarboxylase genes were differentially expressed under acid and osmotic stress conditions (Fig. 4a and Supplementary Fig. 1d ). To identify the precise pathways, we compared mRNA levels of genes encoding glutamate decarboxylase ( gadB and gadA ), arginine decarboxylase ( speA ), S-adenosylmethionine decarboxylase ( speD ), and ornithine decarboxylase ( speF ) by qRT-PCR in the wild-type and ompR null mutant (Fig. 4a and Supplementary Fig. 1a ). The transcript for speF (fivefold) was the most upregulated, compared to speA (1.5-fold) and speD (1.8-fold) in the ompR null strain at high osmolality, suggesting a repressive role of OmpR (Fig. 4a ). In S . Typhimurium, speF levels were identical between the wild-type and ompR null strain, indicating the differing response by OmpR in S . Typhimurium (RpoS repression of yghA ) and E. coli ( speF ) in response to osmotic stress (Figs. 3 and 4b ). Fig. 4 OmpR represses speF to acidify E. coli during osmotic stress. a mRNA levels at pH e 7.2 containing 15% (w/v) sucrose of cadA, cadB, speA, speD, speF, gadA, gadB , and ompF genes were determined by qRT-PCR from wild-type and ompR null strains of E. coli MG1655. Fold expression changes were compared to the wild-type level. The error bars represent the mean ± s.d. ( n = 6). The ompR null strain showed increased transcription of speF at high osmolality. b speF mRNA level of an ompR null strain of S . Typhimurium was compared to the wild-type level at pH e 7.2 in the presence of 15% sucrose (w/v). c Representative R 488/440 images of wild type, an ompR null strain, an ompR / speF null strain, a speF null strain, and the speF over-expressed strain of E. coli grown at pH e 5.6 or pH e 7.2 in the presence of 15% (w/v) sucrose at the indicated time points. Scale bar, 3 μm. d Plot of the R 488/440 ratios of various mutants of E. coli . The complete graph including all strains is in Supplementary Fig. 6 . Data set is represented as the mean ± s.e.m. ( n = 3). e EMSAs were conducted with biotin end-labeled speF to detect OmpR– speF interaction. Lane 2.1* contained 100-fold excess unlabeled DNA Full size image Following osmotic stress, the cadBA (Fig. 1c, d ), gadBA , speA , and speD overexpression strains all acidified to an extent indistinguishable from wild type, whereas the strain over-expressing speF did not acidify (Fig. 4c, d and Supplementary Figs. 1c , d and 6 ). This result identified speF as the predominant decarboxylase that functioned to eliminate protons during osmotic stress to maintain pH homeostasis in E. coli . Overexpression of speF in response to acid stress did not affect the cellular response to acid stress (Fig. 4c, d and Supplementary Fig. 6 ), emphasizing again that the acid and osmotic pathways were distinct. As expected, OmpR was not required for acidification in the absence of speF , and the speF null strain remained similarly acidified compared to the wild type. OmpR bound to the speF regulatory region, as evident from an EMSA (Fig. 4e ). Thus, in E. coli , OmpR represses the speF system to prevent recovery from acidification during osmotic stress. Phosphorylation of EnvZ-OmpR is pH sensitive When the cytoplasm was acidified from either acid or osmotic stress, OmpR was “activated”, leading to repressive effects on transcription at cadC/BA , speF , or rpoS (Figs. 1 – 4 ). We suspected that EnvZ-OmpR phosphorylation might be pH sensitive, as the histidine phosphorylation site must be unprotonated to act as a nucleophile toward ATP [29] . S . Typhimurium or E. coli EnvZ was phosphorylated with [γ- 32 P]-ATP and the percentage of EnvZ~P was determined by densitometry (Fig. 5a ). EnvZ phosphorylation in S . Typhimurium was less robust (70%) than E. coli EnvZ (100%). At pH 5.5, EnvZ phosphorylation was substantially lower when compared to phosphorylation at pH 7.5 for E. coli (28%) and S . Typhimurium (12%), raising the question as to how does activation of OmpR occur during acid and osmotic stress? Fig. 5 OmpR regulation of intracellular pH is non-canonical. a Phosphorylation of EnvZc is acid sensitive. Phosphorylation of E. coli EnvZc compared with S. Typhimurium EnvZc at pH 7.5 and 5.5. The indicated reaction times are above the panel and the percent phosphorylation (determined by densitometry) is listed below. b Representative epifluorescence ratio images (R 488/440 ) were obtained for wild type, an ompR null, an envZ null strain, and the envZ null complemented with envZc (encoding the cytoplasmic domain of EnvZ), and an envZ null complemented with envZcC277Y in S . Typhimurium. Cells were incubated at either acidic pH e 5.6 or pH e 7.2 in the presence of 15% (w/v) sucrose. Scale bar, 3 µm. c A plot of the intracellular pH of 50 cells of wild-type and S . Typhimurium mutants at each indicated time point. Error bars represent the mean ± s.e.m. ( n = 3). d , e OmpR binding to DNA is pH sensitive. AFM images of the 700 bp ompC promoter ( ompC 700 ) from d S . Typhimurium and e E. coli with 30 nM OmpR at acid pH and at neutral pH (the pH used was from the measured values in Fig. 1 ), 30 nM OmpR~P (phosphorylated by acetyl phosphate), and 30 nM (EnvZc + OmpR) at different pH e values. The lengths of the ompC promoter in S . Typhimurium and E. coli were similar (Supplementary Fig. 9h, i ) Full size image Acidification does not require OmpR phosphorylation Canonically, response regulators are phosphorylated by their cognate kinases and phosphorylation drives dimerization. The phosphorylated dimer is an active complex that binds DNA with high affinity and interacts with RNA polymerase to activate transcription. However, some orphan response regulators that lack cognate kinases activate transcription without phosphorylation by mimicking an active interface via dimerization [30] ; (see ref. [11] for a recent review). We reasoned that there might be an acid-dependent conformational change in OmpR that was independent of phosphorylation. We also knew from our previous measurements that EnvZc had higher affinity for OmpR compared to OmpR~P [31] , [32] , which would promote an interaction. We measured the cytoplasmic pH of S . Typhimurium in response to acid and osmotic stress in a D55A OmpR mutant that was incapable of phosphorylation [33] in the presence of the EnvZ kinase. Cytoplasmic acidification occurred in the D55A mutant background in response to either acid or osmotic stress, indicating that OmpR phosphorylation was not required for acidification (Supplementary Fig. 7a, b ). Intriguingly, this phosphorylation-independent activation was completely dependent on the presence of the EnvZ kinase [2] . We therefore examined whether an EnvZ mutant that was incapable of interacting with OmpR (EnvZc C277Y) [10] was still capable of acid-dependent OmpR repression (Fig. 5b, c ). In the presence of the EnvZc C277Y mutant, the S. Typhimurium cytoplasm was no longer acidified in response to acid stress (Fig. 5b, c ). Thus, OmpR must interact with EnvZc to repress CAD, even though phosphoryl transfer was not involved. Gel filtration profiles of EnvZc, EnvZc C277Y, OmpR, (OmpR + EnvZc), and (OmpR + EnvZc C277Y) established that in isolation, both wild-type EnvZc and the EnvZc C277Y mutant existed as dimers, whereas OmpR was monomeric (Supplementary Fig. 8a, b ). In the presence of wild-type EnvZc, OmpR addition generated a higher molecular weight complex, representing two OmpR molecules bound to an EnvZc dimer (Supplementary Fig. 8a ). OmpR dimerization upon interaction with an EnvZc dimer is in agreement with our previous findings using fluorescence cross-correlation spectroscopy [10] . Addition of OmpR to the EnvZc C277Y mutant generated profiles that were identical to the individual proteins in isolation, i.e., no interacting complex was evident (Supplementary Fig. 8b ) and ref. [10] . OmpR is unusual among response regulators, because it can bind DNA in the absence of phosphorylation [34] , presumably because some percentage of the OmpR population exists in an activated, dimeric state. We thus examined whether the oligomeric state of OmpR was affected by acidic conditions (Supplementary Fig. 8c ). The percentage of OmpR dimers increased substantially (to 63–73%), compared to neutral pH, where dimers were undetectable (Supplementary Fig. 8c ). Thus, acid pH can also drive an OmpR conformational change that results in unphosphorylated OmpR dimers. In vivo, this process is driven by interaction with its kinase EnvZ. Acid pH stimulates OmpR binding to DNA How does acidification affect OmpR/DNA interactions? Most DNA-binding assays are sensitive to acidic pH [34] , [35] . For this reason, we turned to AFM to visualize OmpR interactions with the ompC promoter of S. Typhimurium (Fig. 5d ) and E. coli (Fig. 5e ) or the cadBA promoter (Supplementary Fig. 9 ). OmpR was added to a solution buffered to an identical pH i that we measured during acid stress (Fig. 1 ), indicated in the panels. Acid pH alone did not stimulate OmpR aggregation, as evident in the panels that contain OmpR protein in the absence of DNA (Supplementary Fig. 9a ). Addition of OmpR at pH 6.1 ( S . Typhimurium) led to an increase in binding to DNA, compared to addition of OmpR at pH 6.8 (Fig. 5d and Supplementary Fig. 9b ). At pH 6.8, a localized binding of OmpR to ompC DNA was visible as specific, discrete foci (see Supplementary Fig. 9d for quantitation of binding and other controls). Addition of OmpR~P prepared from acetyl phosphate phosphorylation was in-between the level of binding observed at pH 6.8 and 6.1 (Fig. 5d ). A similar stimulation of OmpR binding to DNA in acidic conditions was also evident in E. coli (Fig. 5e and Supplementary Fig. 9c, f ), although the level of acidification was less (6.5 vs. 6.1). In the presence of EnvZ, acidic conditions further increased OmpR binding to the ompC promoter compared to OmpR alone (Fig. 5d, e ; right panels, and Supplementary Fig. 9e, g ). The simplest interpretation of this result is that in vivo, acid pH promotes an activating conformation of EnvZ [9] , [36] that promotes interaction with OmpR, inducing an OmpR conformational change that stimulates dimer formation and favors OmpR binding to DNA. This process is stimulated by OmpR contact with EnvZ, in an interaction that does not involve phosphorylation. Thus, an EnvZ- and acid-dependent conformational change is sufficient to stimulate OmpR binding to DNA (see “Discussion” section). How to reconcile our results with previous studies Our results with the I-switch and BCECF-AM in E. coli and S. Typhimurium (this work and ref. [2] ) differ from previously published studies on the response of E. coli [18] , [37] and S. Typhimurium [38] , [39] to acid stress using pHluorin, a pH-sensitive fluorophore. In addition to using a different fluorophore, some measurements were performed in media with poor buffering capacity using HCl to initiate acid stress. We lowered the pH e of M63 media supplemented with casein hydrolysate from 7.5 to 5.5 by adding 8.5 mM HCl and measured the pH i of E. coli using a similar acid-induction strategy, but measured the response with BCECF-AM and fluorescence microscopy as before. In both S . Typhimurium and E. coli , the cytoplasm was acidified, indicating that the differing results were not a result of different stress conditions (Supplementary Fig. 10a, b ). Plasmid expression of pHluorin is heterogeneous We next examined whether differences were due to the use of different fluorophores. Most previous studies measured the average fluorescence of cultures in solution, whereas our measurements were performed in single cells. We transformed S. Typhimurium and E. coli with ratiometric pHluorin (pH-sensitive GFP) and examined single cells by confocal microscopy after acid or osmotic shock (Fig. 6a ). It was immediately apparent that the cells were extremely heterogeneous with respect to pH values in both S. Typhimurium and E. coli . In fact, in many of the cells, there was no apparent response to acid stress, while in others, there was acidification, but to varying levels. If one determined the average pH of this population in solution, it might very well appear to have “recovered” from acid stress. This level of heterogeneity was not observed in single cells using BCECF-AM (this work) or using the I-switch [2] . Thus, expressing pHluorin using the arabinose-inducible pBAD promoter is not a good indicator for measuring intracellular pH, because it is not uniformly distributed [40] . Constitutive expression of pHluorin was homogeneously distributed, but the fluorescence signal was weak, as previously reported [41] . Fig. 6 Spurious results from using pHluorin, MC4100, and clamping agent sodium benzoate. a S. Typhimurium and E. coli strains harboring a plasmid containing pH-sensitive gfp (pHluorin) exhibit heterogeneity in pH i . Representative epifluorescence (R 405/488 ) ratio images of emission channel 525 nm upon 405 nm excitation and 488 nm excitation were obtained for wild-type cultures at either acidic pH e 5.6 or neutral pH e 7.2. Using ImageJ software, the ratio images were color coded with blue (ratio = 0.1) to white (ratio = 1). Scale bar, 3 µm. The pH of individual cells after 30 min is indicated in the panel. b Representative epifluorescence ratio images (R 488/440 ) were obtained for wild-type cultures of E. coli MC4100 incubated at pH e 5.6, pH e 7.2, and pH e 7.2 with 15% (w/v) sucrose at the indicated times. Scale bar, 3 µm. c A plot of the intracellular pH of 50 cells incubated under acid and osmotic stress conditions at each indicated time. Error bars represent mean ± s.e.m. ( n = 3). d Cells were clamped by either 40 μM nigericin or 30 mM sodium benzoate and the R 488/440 ratio intensities were plotted as a function of pH and overlaid on their in vitro calibration curve. Intracellular pH values determined from BCECF flluorescence of e E. coli MG1655 and f MC4100 clamped with sodium benzoate at pH e 5.6, pH e 6.1, and pH e 7.2 were plotted Full size image MC4100 does not acidify during acid or osmotic stress Another explanation for the differences might be that different strains were employed. We used the sequenced E. coli strain MG1655 [15] , whereas many previous studies used MC4100 [17] . We measured the response of MC4100 to acid stress, using our approach (Fig. 6b, c ). MC4100 was slightly acidified initially compared to MG1655 (pH 6.80 vs. 7.13, respectively), which was comparable to the pH i of S . Typhimurium (Figs. 1 and 6 ). In response to pH e 5.6, E. coli MC4100 maintained its cytoplasmic pH (pH i = 6.83) throughout the experiment (Fig. 6b, c ). The pH i remained essentially unchanged whether the pH e was 7.2, 5.6, or induced by 15% (w/v) sucrose (Fig. 6b, c and Supplementary Fig. 10a, b ). In contrast, addition of osmolytes actually increased the pH i (from 6.8 to 7.15), as reported [18] . This result was opposite to what we observed with E. coli MG1655. Cytoplasmic acidification in the non-pathogenic E. coli Nissle 1917, a widely used probiotic strain [14] , was comparable to E. coli MG1655 and S . Typhimurium (Supplementary Fig. 10d ). Sodium benzoate is not a good clamping agent Most significantly, previous studies generated a standard curve using uncouplers that were reported to collapse ΔpH [6] , [17] , [18] , [38] , [39] . Sodium benzoate was commonly employed for this purpose. Unfortunately, sodium benzoate was not effective at setting pH e = pH i (Fig. 6d ); the standard curve differed dramatically from curves generated from nigericin clamping. To examine this issue further, we used BCECF-AM to measure the pH i of E. coli MG1655 in response to various external pH conditions in the presence of 30 mM sodium benzoate. It was evident that at pH e = 5.6, the pH i was 6.3; at pH e = 6.0, the pH i was 6.2 and at pH e = 7.2, the pH i was 5.8 (Fig. 6e ). Thus, using sodium benzoate at neutral pH e , the intracellular pH would be presumed to have been neutralized, when it was actually quite acidic. These values were not strain dependent, i.e., they were similar for MC4100 and MG1655 (Fig. 6e, f ). Thus, it was evident that sodium benzoate was not an effective clamping agent. This finding also explains why previous measurements of S. Typhimurium pH were substantially different from ours [38] , [39] and why E. coli was reported to return to a neutral pH i [6] , [17] , [18] after an acid stress. More recent measurements in S. Typhimurium using our methods (although not performed in single cells) [42] now are in keeping with our previous findings [2] . The results presented herein establish a new paradigm for pH regulation in Gram-negative bacteria such as E. coli and S . Typhimurium (Fig. 7 ). In contrast to the prevailing view, we determined that E. coli and S . Typhimurium do not recover (within 90 min) due to the repressive actions of OmpR. In both S . Typhimurium and E. coli , OmpR represses the CAD system to acidify the cytoplasm during acid stress (Fig. 1 ). In S . Typhimurium, the pathway for acidification during osmotic stress involves rpoS and the putative oxidoreductase YghA. Increasing YghA expression (via OmpR repression of rpoS ), increased proton production, which acidified the cytoplasm. In E. coli , OmpR repressed speF (which consumes protons) during osmotic stress (Fig. 5 and model, Fig. 7 ). Fig. 7 Model for OmpR-driven acidification in response to acid and osmotic stress. Under acid and osmotic stress conditions, both S . Typhimurium and E. coli are acidified in an OmpR-dependent manner. OmpR requires interaction with EnvZ, but not phosphorylation to bring about cytoplasmic acidification. a In wild-type bacteria, under acid stress, OmpR represses the cad operon to eliminate proton consumption, resulting in acidification. At high osmolality, in S . Typhimurium, OmpR represses rpoS to relieve rpoS repression of yghA , producing protons. In E. coli , OmpR represses ornithine decarboxylase ( speF) , enabling cytoplasmic acidification. The pH optima of CadA is 6.1–6.5 [21] , this optima contributes to a threshold of response. At pH 6.5 and below (achieved during acid stress), OmpR represses the cad operon, resulting in acidification. At high osmolality (pH 6.75 E. coli , 6.45, S. Typhimurium), acidification is less, because the CAD system is working to restore neutrality. Acidification occurs through proton production ( S. Typhimurium) or repression of a different amino acid decarboxylation system ( E. coli ). Intracellular acidification is required for activating SPI-2-dependent effector secretion. EnvZ senses and responds to cytoplasmic acidification via helix-coil transitions. A physical interaction of OmpR with EnvZ drives a conformational change, resulting in unphosphorylated OmpR dimer formation. EnvZ-dependent OmpR dimerization creates an active OmpR 2 interface, favoring DNA binding and subsequent repression. b In the ompR null strain, during acid stress, CadC/BA is expressed, and drives amino acid decarboxylation. This process consumes intracellular protons, restoring cytoplasmic pH and maintaining intracellular pH homeostasis. At high osmolality, in an ompR null S . Typhimurium strain, RpoS represses yghA , preventing proton release, resulting in a neutralized cytoplasm. In an ompR null E. coli strain, activated SpeF eliminates cytoplasmic protons during ornithine decarboxylation, maintaining pH homeostasis Full size image Our results indicate that EnvZ functions to sense acidic pH in the cytoplasm, resulting from extracellular acid or osmolytes (Figs. 1 and 2 ). Although OmpR was capable of repressing genes in the absence of phosphorylation, EnvZ was required. We interpret this result in the following way: acidification promotes helicity [36] ; EnvZ responds to cytoplasmic signals by increased helicity of the 17 amino acid region surrounding the phosphorylated histidine [9] . Phosphorylation was slow at acid pH (Fig. 5a ), but a physical interaction of OmpR with EnvZ promoted dimerization (Fig. 5b, c and Supplementary Fig. 8a, b ), creating an active OmpR 2 interface that bound DNA with higher affinity (Fig. 5d, e ). With an isoelectric point of OmpR at 6.04, its conformation is exquisitely sensitive to changes in cytoplasmic acidity. The present work identifies a critical pH threshold in bacteria that establishes a signaling node. In Salmonella , acidification to pH 6.1 leads to OmpR repression of CAD (Fig. 1 ) and activation of SPI-2 gene expression, as evident by increasing ssrB transcription and SseJ effector secretion (Supplementary Fig. 3 ). E. coli is acidified to pH 6.55, again via OmpR repression of CAD. Osmolytes also lead to acidification, but only to ~pH 6.45 ( Salmonella ) or 6.75 ( E. coli ) (Fig. 1 ). The cytoplasm is less acidic during osmotic stress due to the competing effects of CAD activation (Fig. 4 ) and relief of rpoS repression leading to yghA activation in Salmonella , or speF repression in E. coli . This threshold likely is set by the level of OmpR “activation” and perhaps the effects of acid pH on its conformation. The activated state of OmpR is influenced by numerous factors, including a physical interaction with EnvZ (Fig. 5b, c and Supplementary Fig. 8a, b ), phosphorylation [35] , [43] , dimerization (Supplementary Fig. 8a, b, c ), and an acid-dependent effect on OmpR conformation (Fig. 5d, e ). We are presently exploring the effect of acid pH on OmpR conformation by NMR to determine whether effects of acid pH differ from or are similar to the effect of EnvZ on OmpR conformation. Most significantly, the present work highlights that the method for setting pH e = pH i using sodium benzoate actually produces the opposite effect. At a neutral external pH, addition of sodium benzoate substantially acidified both S. Typhimurium and E. coli (Fig. 6 ). This finding, we believe, accounts for the substantial differences between our studies and the published literature. This study provides evidence for a new view of the response to acid/osmotic stress in bacteria and emphasizes the intriguing differences in prokaryotes compared to eukaryotes, where intracellular pH and osmolality are tightly regulated. A deeper understanding of these differences will provide new approaches for combating the virulence strategies employed by pathogens to survive in acid environments and secrete virulence factors. Bacterial strains, antibodies, and growth conditions S enterica . serovar Typhimurium 14028s and E. coli MG1655 were used in this study unless otherwise indicated. To determine the acid and osmotic stress response, bacterial strains were grown in a modified N-minimal medium (MgM) buffered with 100 mM Tris (pH 7.2 ± 15% (w/v) sucrose) or 100 mM MES (pH 5.6) as described [2] . The casamino acids included in the media provided sufficient lysine for activation of the CAD system. The following antibodies were used for immuno-labeling experiments: rabbit polyclonal anti-HA (catalog no. S190–108, Axil Scientific) 1:5000, anti-rabbit secondary antibody (catalog no. SC-2357, Santa Cruz) 1:5000. Ampicillin was used at 100 µg ml −1 , chloramphenicol at 30 µg ml −1 , kanamycin 30 µg ml −1 , and tetracycline at 12.5 µg ml −1 . For clamping experiments, bacteria were incubated at various external pH values with either nigericin (40 µM) or sodium benzoate (30 mM) at RT for 1 h. Overnight wild-type cultures of S. Typhimurium and E. coli in LB-expressing pHluorins were subcultured into fresh LB in the presence of 0.2% L-arabinose for 2 h (OD ~0.25). The cultures were then centrifuged and incubated in MgM media at either acidic pH e 5.6 or neutral pH e 7.2 containing 0.2% L-arabinose. The intracellular pH was measured every 30 min for 3 h (OD ~0.8). Wide-field fluorescence and confocal microscopy For pH measurements using BCECF-AM, wide-field images were collected using an Olympus IX71 Inverted Microscope (Applied Precision DeltaVision Deconvolution microscope system) equipped with ×100, 1.4 numerical aperture objective lens. Image capture was performed with the CoolSnap HQ, a fast, high-resolution, high-quantum efficiency, cooled CCD camera (Photometrics CoolSNAP HQ2 (CCD); 1392 × 1040 pixels; 11 fps). Two channels were selected for acquiring paired sets of images corresponding to emission wavelength (525/36 nm) upon donor excitation of either 490 ± 20 nm (pH-sensitive wavelength), or 436 ± 10 nm (pH-insensitive wavelength). Both channels had the same exposure time of 10 s. The emission ratios upon excitation (490/436) were obtained by using the ratio plus plug-in of ImageJ software version 1.42. The ratios were plotted as a function of pH, and were comparable to the in vitro calibration curve. The high and low values were color coded and calibrated to their respective pH values as described in ref. [2] . For pH measurements using pHluorin, confocal imaging was conducted on an inverted Nikon A1Rsi-Polarizing Module equipped with CFI Plan ApochromatVC ×100, 1.4 numerical aperture objective lens using Coherent CUBE lasers at 405 and 488 nm excitation with set appropriate dichroics. Sequential scans were performed to obtain paired set of images by using excitation wavelengths of either (405 ± 30 nm) or (470 ± 40 nm) and the emission was recorded through a 525/50 nm band pass filter on a Andor DU897 EMCCD camera. The ratiometric images were obtained by dividing the emission at excitation 405 by 470 nm and analyzed using the ratio plus plug-in of ImageJ version 1.42. High and low values were color coded and calibrated to their respective pH values. Measurement of BCECF in S . Typhimurium and E coli Cultures of S . Typhimurium and E. coli were pre-incubated with 20 μM BCECF-AM for 60 min before the shift to acidic pH e (5.6), neutral pH e (7.2), or high osmolality pH e 7.2 plus 15% (w/v) sucrose. Cell-permeant BCECF incorporation into cells is evident from the fluorescent images. Cells were then washed with the incubation media to eliminate extracellular BCECF prior to imaging. Ratios of fluorescence intensities of the emission channel (525 nm) upon 488 nm excitation and 440 nm excitation were obtained and compared to the in vitro standard curve as described above and in ref. [2] . Cells were placed on microscope slides (Marienfeld) coated with 1% (w/v) agarose and images were analyzed by ImageJ version 1.42. Construction of mutants and overexpression strains Chromosomal copies of yghA and rpoS from wild-type or an ompR null strain of S . Typhimurium and cadBA , speF from wild-type or an ompR null strain of E. coli were replaced by tetRA using λ-Red recombination techniques [44] . To generate an ompR/yghA/rpoS null strain of S. Typhimurium, a Cm R cassette amplified from plasmid pKD3 using primers yhgA: : Cm #1F and yhgA: : Cm #1R was integrated into an ompR/rpoS double null strain. The rpoS , speA , speD, speF , gadBA , yghA , and cadBA over-expressed strains were generated by cloning the genes into pBR322 by replacement of bla [2] . The pH-sensitive gfp (“pHluorin”) gene was cloned into plasmid pMPM - A5omega and placed under control of the arabinose -inducible pBAD promoter. OmpR site-specific mutant D55 (primers D55AF/D55AR) and EnvZ site-specific mutant C277Y (primers C277YF/C277YR) were introduced following the QuikChange® Site-Directed Mutagenesis Kit (Stratagene) and substitutions were verified by DNA sequencing. 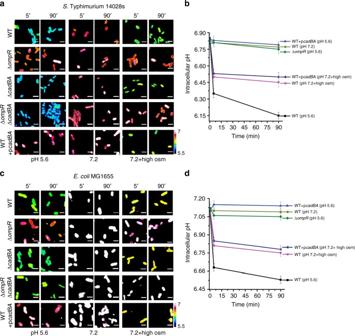Fig. 1 OmpR drives intracellular acidification in response to acid stress.a–dS. Typhimurium andE. colicultures were incubated with 20 µM BCECF for 60 min before imaging. Representative epifluorescence ratio images (R488/440) of emission channel 525 nm upon 488 nm excitation and 440 nm excitation were obtained for wild type, anompRnull mutant, anompR/cadBAnull strain, acadBAnull strain, and acadBAover-expressed strain ofaS. Typhimurium andcE. coliincubated at either acidic pHe(5.6) or neutral pHe(7.2) or at pHe(7.2) plus 15% (w/v) sucrose. Using ImageJ software, ratio images were color coded with blue (ratio = 0.1) to white (ratio = 1). Scale bar, 3 µm. A plot of the intracellular pH of 50 cells of wild type and mutants ofbS. Typhimurium anddE. coliat each indicated time point. Error bars represent the mean ± s.e.m. (n= 3). The complete graphs including all strains inb,care in Supplementary Fig.2. Repression of thecadoperon was not responsible for intracellular acidification during osmotic stress inS. Typhimurium andE. coli The strains are listed in Table 1 and the primers used are in Supplementary Table 1 . Table 1 Strains and plasmid used in this study Full size table Electrophoretic mobility shift assay EMSAs were performed using the Lightshift chemi-luminescence EMSA kit (Research instruments) according to the manufacturer’s instructions as described [2] . Upstream regions of E. coli cadB (347 bp), cadA (350 bp), speF (384 bp), and S . Typhimurium rpoS (420 bp) and yhgA (370 bp) were amplified using biotinylated oligonucleotides. Ten fmol of biotinylated DNA was used in a 15 μl reaction containing binding buffer (10 mM Tris, pH 7.5, 50 mM KCl) along with 2.5% (w/v) glycerol, 1 mM MgCl 2 , 0.05% (w/v) Nonidet P-40, and 1 μg poly(dI-dC). This interaction was specific, as addition of a 100-fold excess of unlabeled DNA was added to examine specific interaction (labeled *). OmpR or OmpR~P protein was added at the concentrations indicated, and samples were separated by electrophoresis on 5% non-denaturing acrylamide gels run in 0.5× Tris-acetate buffer with EDTA. RNA isolation and qRT-PCR E. coli and S . Typhimurium strains were grown in MgM media at pH 5.6, 7.2, and 7.2 with 15% (w/v) sucrose to OD ~0.6 as described [2] . Total RNA was isolated, followed by cDNA synthesis and quantification. The mRNA expression level of the target gene was normalized relative to 16S rRNA. Western blot with anti-SseJ antibody Total and secreted protein fractions were isolated from wild type and an ssaJ null strain of S . 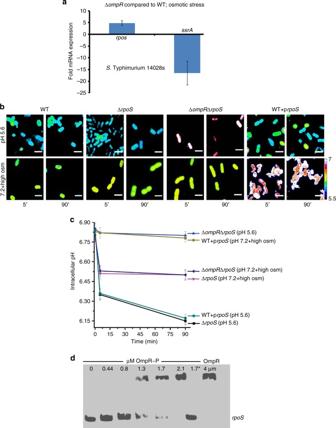Fig. 2 Osmotic stress acidifiesS.Typhimurium via OmpR repression ofrpoS.amRNA levels ofrposandssrA(a positive control) genes were determined by qRT-PCR from wild-type andompRnull strains ofS. Typhimurium grown at high osmolality. Fold expression changes in theompRnull strain was compared to the wild-type level and plotted. The error bars represent the mean ± s.d. (n= 6). In theompRnull strain,rpoStranscription was increased, suggesting OmpR repression.bRepresentative images of R488/440are shown after 5 and 90 min incubation at pHe7.2 or pHe7.2 in the presence of 15% (w/v) sucrose (high osm) of wild type, anompR/rpoSnull strain, anrpoSnull strain, and anrpoSover-expressed strain ofS. Typhimurium. Scale bar, 3 μm.cA plot from 50 cells of the R488/440ratios of various mutants ofS. Typhimurium at indicated times. Symbols represent the mean ± s.e.m. (n= 3).dAn EMSA examined the interaction between OmpR andrpoS. OmpR was incubated with 10 fmol of biotin end-labeledrpoS. Lane 1.7* contained 100-fold excess unlabeled DNA Typhimurium harboring p sseJ -HA. Protein samples were separated by 10% SDS-PAGE followed by transfer to a PVDF membrane. The membrane was incubated with anti-HA (1:5000) or anti-GroEL (1:5000) and a secondary anti-HA HRP antibody (1:5000) was used for detection. Overexpression and purification: OmpR, EnvZc, and EnvZc C277Y E. coli BL21 (DE3) was used for overproduction of full-length His-OmpR cloned into pET15b as described [34] , [45] . Purified OmpR was buffer exchanged (i.e., 20 mM Tris with 200 mM NaCl) buffered at pH 6.1, 6.5, 6.8, or 7.2, and the purity was examined by SDS-PAGE. S . Typhimurium and E. coli EnvZc were subcloned into pET28b, over-expressed and purified as in ref. [45] . Overexpression and purification of S. Typhimurium EnvZc C277Y protein was as described for wild-type EnvZc. Atomic force microscopy Seven hundred base pair regions from ompC (−607 to +93 bp), cadB (−673 to +27 bp), and yghA (−673 to +27 bp) were gel-purified using the QIAquick Gel Extraction Kit (Qiagen). A glutaraldehyde-modified mica surface was prepared as described [46] . Ten nanogram of the regulatory region was incubated with 30 nM OmpR or OmpR~P (prepared by phosphorylation from acetyl phosphate [35] at pH 5.6 or 7.2 ± 15% (w/v) sucrose for 15 min at RT. 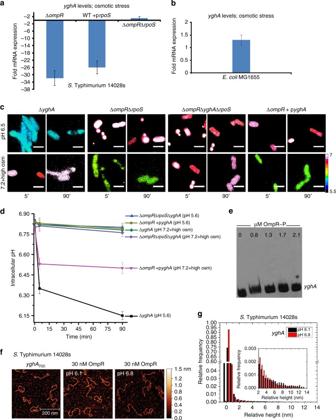Fig. 3 OmpR relieves RpoS repression ofyghAduring osmotic stress.amRNA levels ofyghAat pHe7.2 in the presence of 15% sucrose (w/v) were determined by qRT-PCR from wild type, anompRnull strain, anrpoSover-expressed strain, and anompR/rpoSnull strain ofS. Typhimurium. Fold expression changes were compared to the wild-type level. Error bars represent the mean ± s.d. (n= 6).bmRNA ofyghAat pHe7.2 in the presence of 15% sucrose (w/v) of anE. coli ompRnull strain was compared to the wild-type level.cRepresentative images of R488/440are shown after 5 and 90 min incubation at pHe5.6, or pHe7.2 + 15% (w/v) sucrose of ayghAnull strain, anompR/rpoSnull strain, anompR/rpoS/yghAnull strain, and anompRnull strain ofS.Typhimurium withyghAover-expressed. Scale bar, 3 μm.dPlot of the R488/440ratios of various mutants ofS.Typhimurium at each indicated time. Data set is represented as the mean ± s.e.m. (n= 3). The complete graph, including all strains is in Supplementary Fig.4.eEMSAs were performed with biotin end-labeledyghAand OmpR.fAFM images ofyghA700fromS. Typhimurium with 30 nM OmpR at either acid pH (6.1) or neutral pH (6.8).gRelative height distribution histogram of theyghApromoter complexed with 30 nM OmpR at either acidic or neutral pH 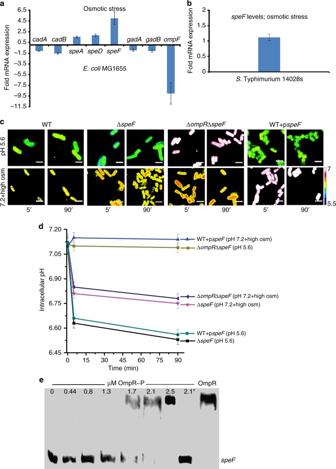Fig. 4 OmpR repressesspeFto acidifyE. coliduring osmotic stress.amRNA levels at pHe7.2 containing 15% (w/v) sucrose ofcadA, cadB, speA, speD, speF, gadA, gadB, andompFgenes were determined by qRT-PCR from wild-type andompRnull strains ofE. coliMG1655. Fold expression changes were compared to the wild-type level. The error bars represent the mean ± s.d. (n= 6). TheompRnull strain showed increased transcription ofspeFat high osmolality.bspeFmRNA level of anompRnull strain ofS. Typhimurium was compared to the wild-type level at pHe7.2 in the presence of 15% sucrose (w/v).cRepresentative R488/440images of wild type, anompRnull strain, anompR/speFnull strain, aspeFnull strain, and thespeFover-expressed strain ofE. coligrown at pHe5.6 or pHe7.2 in the presence of 15% (w/v) sucrose at the indicated time points. Scale bar, 3 μm.dPlot of the R488/440ratios of various mutants ofE. coli. The complete graph including all strains is in Supplementary Fig.6. Data set is represented as the mean ± s.e.m. (n= 3).eEMSAs were conducted with biotin end-labeledspeFto detect OmpR–speFinteraction. Lane 2.1* contained 100-fold excess unlabeled DNA This mixture was then deposited on the mica for 15 min. Images were acquired on a Bruker Dimension FastScan AFM system using the tapping mode with a silicon nitride cantilever (FastScan C, Bruker). Raw AFM images were processed using Gwyddion software ( http://gwyddion.net/ ). Gel filtration chromatography Gel filtration chromatography was carried out on a Hiload 16/60 Superdex 75 pg (Amersham Biosciences) and Superose ® 12 10/300 GL (Sigma-Aldrich) size exclusion chromatography columns for OmpR and EnvZc, respectively, on an AKTA FPLC system (Amersham Biosciences) using suitable buffers. 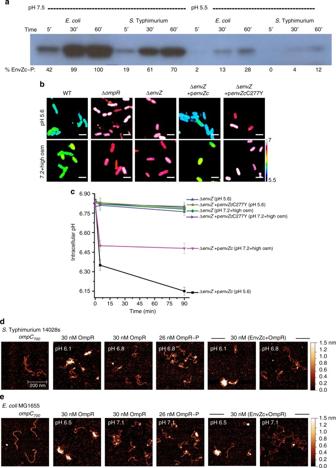Fig. 5 OmpR regulation of intracellular pH is non-canonical.aPhosphorylation of EnvZc is acid sensitive. Phosphorylation ofE. coliEnvZc compared withS.Typhimurium EnvZc at pH 7.5 and 5.5. The indicated reaction times are above the panel and the percent phosphorylation (determined by densitometry) is listed below.bRepresentative epifluorescence ratio images (R488/440) were obtained for wild type, anompRnull, anenvZnull strain, and theenvZnull complemented withenvZc(encoding the cytoplasmic domain of EnvZ), and anenvZnull complemented withenvZcC277YinS. Typhimurium. Cells were incubated at either acidic pHe5.6 or pHe7.2 in the presence of 15% (w/v) sucrose. Scale bar, 3 µm.cA plot of the intracellular pH of 50 cells of wild-type andS. Typhimurium mutants at each indicated time point. Error bars represent the mean ± s.e.m. (n= 3).d,eOmpR binding to DNA is pH sensitive. AFM images of the 700 bpompCpromoter (ompC700) fromdS. Typhimurium andeE. coliwith 30 nM OmpR at acid pH and at neutral pH (the pH used was from the measured values in Fig.1), 30 nM OmpR~P (phosphorylated by acetyl phosphate), and 30 nM (EnvZc + OmpR) at different pHevalues. The lengths of theompCpromoter inS. Typhimurium andE. coliwere similar (Supplementary Fig.9h, i) Two column volumes of running buffer was used to pre-equilibrate, the flow rate was 0.5 ml min −1 . Eluted peaks were quantified by absorbance at 280 nm and fractions were analyzed by SDS-PAGE. Measurement of intracellular NAD + /NADH Intracellular NAD + /NADH levels were determined using an NAD + /NADH assay kit (ProBioscience Technologies) from S . Typhimurium cultures grown for 90 min at acidic pH e (5.6), neutral pH e (7.2), or high osmolality pH e (7.2) plus 15% (w/v) sucrose. Cells were normalized to OD 600 = 0.8 and total NAD + and NADH levels were determined per ml of bacteria. 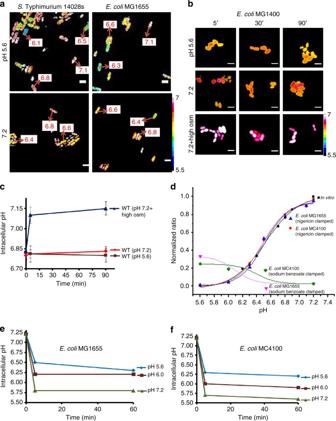Fig. 6 Spurious results from using pHluorin, MC4100, and clamping agent sodium benzoate.aS.Typhimurium andE. colistrains harboring a plasmid containing pH-sensitivegfp(pHluorin) exhibit heterogeneity in pHi. Representative epifluorescence (R405/488) ratio images of emission channel 525 nm upon 405 nm excitation and 488 nm excitation were obtained for wild-type cultures at either acidic pHe5.6 or neutral pHe7.2. Using ImageJ software, the ratio images were color coded with blue (ratio = 0.1) to white (ratio = 1). Scale bar, 3 µm. The pH of individual cells after 30 min is indicated in the panel.bRepresentative epifluorescence ratio images (R488/440) were obtained for wild-type cultures ofE. coliMC4100 incubated at pHe5.6, pHe7.2, and pHe7.2 with 15% (w/v) sucrose at the indicated times. Scale bar, 3 µm.cA plot of the intracellular pH of 50 cells incubated under acid and osmotic stress conditions at each indicated time. Error bars represent mean ± s.e.m. (n= 3).dCells were clamped by either 40 μM nigericin or 30 mM sodium benzoate and the R488/440ratio intensities were plotted as a function of pH and overlaid on their in vitro calibration curve. Intracellular pH values determined from BCECF flluorescence ofeE. coliMG1655 andfMC4100 clamped with sodium benzoate at pHe5.6, pHe6.1, and pHe7.2 were plotted 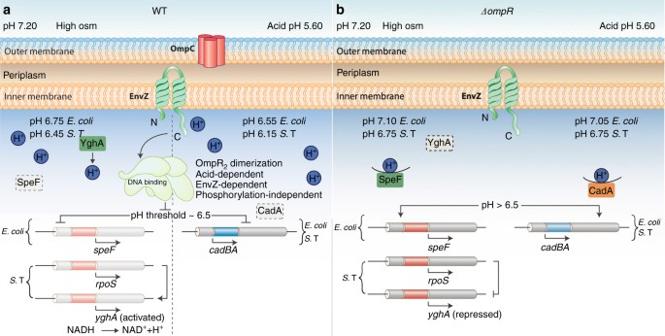Fig. 7 Model for OmpR-driven acidification in response to acid and osmotic stress. Under acid and osmotic stress conditions, bothS. Typhimurium andE. coliare acidified in an OmpR-dependent manner. OmpR requires interaction with EnvZ, but not phosphorylation to bring about cytoplasmic acidification.aIn wild-type bacteria, under acid stress, OmpR represses thecadoperon to eliminate proton consumption, resulting in acidification. At high osmolality, inS. Typhimurium, OmpR repressesrpoSto relieverpoSrepression ofyghA, producing protons. InE. coli, OmpR represses ornithine decarboxylase (speF), enabling cytoplasmic acidification. The pH optima of CadA is 6.1–6.521, this optima contributes to a threshold of response. At pH 6.5 and below (achieved during acid stress), OmpR represses thecadoperon, resulting in acidification. At high osmolality (pH 6.75E. coli, 6.45,S.Typhimurium), acidification is less, because the CAD system is working to restore neutrality. Acidification occurs through proton production (S.Typhimurium) or repression of a different amino acid decarboxylation system (E. coli). Intracellular acidification is required for activating SPI-2-dependent effector secretion. EnvZ senses and responds to cytoplasmic acidification via helix-coil transitions. A physical interaction of OmpR with EnvZ drives a conformational change, resulting in unphosphorylated OmpR dimer formation. EnvZ-dependent OmpR dimerization creates an active OmpR2interface, favoring DNA binding and subsequent repression.bIn theompRnull strain, during acid stress, CadC/BA is expressed, and drives amino acid decarboxylation. This process consumes intracellular protons, restoring cytoplasmic pH and maintaining intracellular pH homeostasis. At high osmolality, in anompRnullS. Typhimurium strain, RpoS repressesyghA, preventing proton release, resulting in a neutralized cytoplasm. In anompRnullE. colistrain, activated SpeF eliminates cytoplasmic protons during ornithine decarboxylation, maintaining pH homeostasis Intracellular NAD + /NADH levels (nM) were converted using NAD + standards of known concentration. Statistical analysis For intracellular ATP, NAD + /NADH, and pH measurements, the results are presented as mean ± s.e.m. For quantification of mRNA levels, it is mean ± s.d. Data availability The microarray data that are available have been deposited with the GEO (accession code: GSE106630). All other relevant data are available from the corresponding author on request.